Real-timein vivoimaging of invasive- and biomaterial-associated bacterial infections using fluorescently labelled vancomycin Invasive and biomaterial-associated infections in humans are often difficult to diagnose and treat. Here, guided by recent advances in clinically relevant optical imaging technologies, we explore the use of fluorescently labelled vancomycin (vanco-800CW) to specifically target and detect infections caused by Gram-positive bacteria. The application potential of vanco-800CW for real-time in vivo imaging of bacterial infections is assessed in a mouse myositis model and a human post-mortem implant model. We show that vanco-800CW can specifically detect Gram-positive bacterial infections in our mouse myositis model, discriminate bacterial infections from sterile inflammation in vivo and detect biomaterial-associated infections in the lower leg of a human cadaver. We conclude that vanco-800CW has a high potential for enhanced non-invasive diagnosis of infections with Gram-positive bacteria and is a promising candidate for early-phase clinical trials. Bacterial infections are of mounting medical and public concern. As human life expectancy continues to increase, so has the number of frail and immune-compromised individuals who are susceptible to bacterial infections. A major contributor to this trend is the proliferation of medical implants and devices, which are inherently vulnerable to bacterial contamination. To complicate matters further, current antimicrobial therapies face challenges from the emergence of omnipresent drug-resistant microbes such as methicillin-resistant Staphylococcus aureus . Infections precipitated by implanted materials occur at high frequency and are difficult to diagnose and treat. For example, ~5% of the inserted internal fixation devices in bone fractures become infected. This number rises to ~30% after fixation of open fractures [1] . Apart from the clinical implications and burden on the patients’ quality of life, the costs for treating such severe complications can be as much as $107,000 per case [2] . A major challenge in averting biomaterial-associated infections (BAIs) is the lack of a sensitive, specific and non-invasive modality to detect early-stage bacterial infections, when treatment is most effective owing to the absence of profound biofilm formation. Currently, only indirect imaging modalities are in clinical use, as exemplified by positron emission tomography with fluoro-deoxy-glucose, which visualizes increased glucose uptake by inflammatory cells [3] . Alternatively, sites of inflammation can be located by injection of radiolabelled leukocytes and subsequent scanning. Unfortunately, these approaches lack sufficient resolution, practicality and cannot clearly discriminate between a bacterial infection and general inflammation. Therefore, clinical imaging tools that are easy-to-use, allow bedside monitoring, and directly target invasive bacteria are highly desirable. Radiolabelled antibiotics are attractive ligands that directly bind to pathogenic bacteria [4] . However, their general use is hampered by inherent limitations in specificity and resolution (~0.5 cm) of the radiologic imaging modality [4] , [5] , [6] , [7] and radioactivity itself. Optical imaging, in particular targeted fluorescent imaging (TFLI), is a relatively novel diagnostic approach that has attracted increasing support for both preclinical and clinical applications. TFLI is based on the administration of an exogenous targeting fluorophore that emits light outside the absorbance window of bodily tissues. Emitted signals are readily detected by a sensitive charge-coupled device camera. Clear advantages of TFLI include the following: (i) non-invasive real-time imaging, (ii) high resolution, (iii) absence of radiation-related risks and (iv) relatively low costs. Animal-based experiments have shown the feasibility of TFLI for detecting tumours. Moreover, the first proof-of-principle study for clinical use of TFLI in ovarian cancer surgery has been recently reported [8] . Recent pioneering studies have demonstrated the feasibility of TFLI for in vivo detection of bacteria [9] , [10] , [11] . Before introducing this approach into the clinic, however, several essential steps need to be carried out, including toxicity testing of the fluorescent probe for its clinical translation, according to international guidelines and standards such as the Good Clinical Practice guidelines ( http://www.ich.org/products/guidelines.html ). With the aforementioned requirements in mind, we propose to use a novel fluorescent imaging agent derived from the drug vancomycin as a diagnostic tool for detecting infecting bacteria in vivo . As vancomycin has been used clinically for over 50 years, there is widespread familiarity with the pharmacokinetics, biodistribution and toxicity profile. For usage as an optical imaging agent to selectively target Gram-positive bacteria in vivo , we conjugated vancomycin to IRDye 800CW, a near-infrared (NIR) fluorophore now in early clinical trial (NCT01508572; Fig. 1a ). Vancomycin is a glycopeptide antibiotic drug that exhibits preferential activity against Gram-positive bacteria, which are the most prominent causative agents of soft tissue infections and BAIs. Vancomycin binds specifically to the D-Ala-D-Ala moiety present in bacterial cell walls ( Fig. 1b ). Biodistribution of a vancomycin-based agent can be similar to that of unlabelled vancomycin, as shown by single photon-emission computed tomography studies in rats [12] . In the present study, we show that NIR optical imaging with a bacteria-specific vancomycin-based probe can detect both invasive infections in vivo and BAIs post mortem . 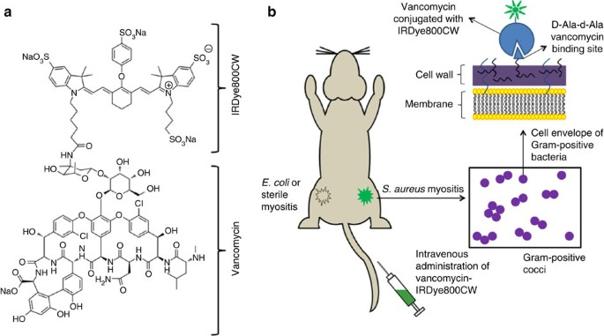Figure 1: Vancomycin-IRDye 800CW and the experimental approach. (a) Structure of vanco-800CW. (b) Schematic representation of the experimental approach for imaging mice injected with eitherS. aureus(S. aureusmyositis),E. coli(E. colimyositis) or Cytodex beads (sterile myositis), and subsequent detection ofS. aureuswith vanco-800CW. Figure 1: Vancomycin-IRDye 800CW and the experimental approach. ( a ) Structure of vanco-800CW. ( b ) Schematic representation of the experimental approach for imaging mice injected with either S. aureus ( S. aureus myositis), E. coli ( E. coli myositis) or Cytodex beads (sterile myositis), and subsequent detection of S. aureus with vanco-800CW. Full size image Detection of clinical bacterial isolates in vitro To determine the binding specificity of vanco-800CW, bacterial isolates from infected orthopaedic material of 19 patients at the University Medical Center Groningen were cultured, incubated with vanco-800CW and subsequently imaged with an IVIS Spectrum. Notably, these isolates form a representative display of the microorganisms encountered in BAIs, including S. aureus , Staphylococcus epidermidis , Corynebacterium species, Streptococcus or closely related bacterial species (Group G Streptococcus species, Streptococcus mitis and Granulicatella adiacens ), Dermabacter hominis , Escherichia coli , Klebsiella species, Enterobacter species and Pseudomonas species. By this ex-vivo fluorescence imaging approach, all of the 18 tested Staphylococcus isolates were detected, and also 21 of the 25 tested Gram-positive bacterial isolates (84%; Supplementary Fig. S1a ) were detected. The Gram-positive isolates with a fluorescent signal below the preset detection limit (that is, intensity: 10 5 net counts) mainly consisted of Corynebacterium species (4/6). In addition, 10 out of 11 Gram-negative bacterial isolates (91%) were undetectable using the above parameters, as expected based on the pharmacological preference of vancomycin for targeting Gram-positive bacteria. To determine the minimal number of bacteria detectable by TFLI, a dilution series was performed using a S. aureus isolate derived from a clinical sample, labelled with vanco-800CW. The bacteria were then counted using a counting chamber. In the dilution series, the minimum fluorescence detection level approximated 1.2 × 10 4 net counts. After incubation with vanco-800CW, ~5 × 10 6 staphylococci were detected in 200 μl, corresponding to 2.5 × 10 4 staphylococci per mm 3 ( Supplementary Fig. S1b ). Bacterial myositis in mice The in vivo applicability of vanco-800CW was subsequently tested in immunocompetent mice that had myositis in the left hind limb induced by intramuscular injection of luciferase-engineered S. aureus . The S. aureus strain’s constitutive bioluminescence facilitates localization of live bacteria by simultaneous imaging of the fluorescence signal derived from vanco-800CW and luciferase bioluminescence. Two days after intramuscular inoculation with S. aureus , six mice were intravenously injected with vanco-800CW (at 0.1, 1, 3 or 5 mg kg −1 , in which 1 mg kg −1 was administered in several mice, as this was the expected optimal targeting dose). After an additional 24 h, both bioluminescence and fluorescence imaging were performed with an IVIS Lumina II imaging system. A strong NIR fluorescence (NIRF) signal, attributed to vanco-800CW, was observed to colocalize with the bioluminescence signal in all administered doses (that is, an intensity of 3.7 × 10 5 ±9.8 × 10 4 counts ex vivo at a dose of 1 mg kg −1 ; Supplementary Fig. S2a ). In addition, the bladder gave a strong signal, which was no longer detectable after draining ( Supplementary Fig. S3a ). No NIRF signal was observed in infected mice that did not receive vanco-800CW. Importantly, in a co-infection experiment wherein mice were injected with luciferase-engineered S. aureus in one hind limb and luciferase-engineered E. coli in the other, a vanco-800CW-specific fluorescent signal was observed only for the staphylococcal myositis ( Fig. 2a ). Ex vivo , the fluorescence signal also colocalized with the bioluminescence signal ( Fig. 2b and Supplementary Fig. S2b ). A significant increase in fluorescence signal was observed for the infected muscle in comparison with the contralateral non-infected hind limb (1.0 × 10 5 ±4.2 × 10 4 counts; P =0.007). Infected tissue yielded a target-to-background (TBR) ratio of 4.2 corrected for background signal, over the non-infected tissue in the contralateral leg ex vivo . Notably, although we observed large overlaps between the bioluminescence and fluorescence signals, the match between both signals was not 100% ( Fig. 2c , Supplementary Fig. S4 and Supplementary Movie 1 ). We attribute this to a combination of factors, including (i) different threshold settings in the bioluminescence and fluorescence imaging; (ii) differences in wavelengths of the light emitted through bioluminescence (luciferin peak at 490 nm) and NIRF (IRDye800CW peak at 800 nm), which result in significantly different tissue scattering and absorption properties; and (iii) the fact that only exponentially growing cells are bioluminescent ( Supplementary Fig. S5 ), whereas staining with vanco-800CW is independent of the growth phase. Fluorescence microscopy demonstrated that the fluorescence in the 800 nm channel was directly related to the presence of vanco-800CW-labelled staphylococci ( Fig. 2d and Supplementary Fig. S6 ), as also detected by Giemsa staining and confirmed by fluorescent in situ hybridization microscopy ( Supplementary Fig. S2c,d ). In contrast, no NIR signal was observed for the E. coli cells ( Fig. 2d and Supplementary Fig. S6 ). Culturing of homogenized infected muscle tissue after macroscopic optical imaging revealed the presence of S. aureus (~6.4 × 10 7 colony-forming units (CFUs)), which was confirmed by ex-vivo bioluminescence imaging. After autopsy, fluorescence signal was also detected in the kidneys, liver and urine of vanco-800CW-treated mice ( Supplementary Figs S3b and S7 ), which is consistent with the strong in vivo bladder signal ( Supplementary Fig. S3a ) and the known pharmacokinetic profiles of unlabelled vancomycin and unmodified IRDye 800CW (both eliminated by the kidneys) [13] , [14] , [15] . The heart, spleen, normal muscle and bowel showed no fluorescence signal above background levels ( Supplementary Fig. S7 ). 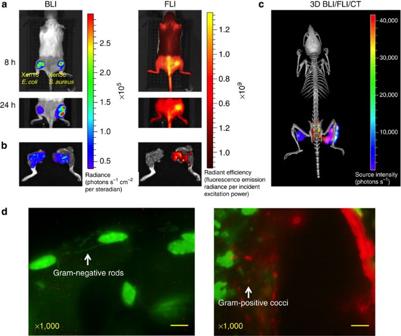Figure 2:In-vivoimaging of bacterial myositis. (a) Imaging of a mouse withE. coli(Xen16)-induced myositis in the left hind limb andS. aureus(Xen36)-induced myositis in the right hind limb was performed with the IVIS SpectrumCT Imaging System at 8 and 24 h after intravenous administration of 1.8 mg kg−1vanco-800CW. Left side: bioluminescence imaging (open filter, field of view (FOV) 12.8 cm, F-stop 1, 30 s acquisition time); right side: fluorescence imaging (excitation 745 nm, emission 840 nm, field of view (FOV) 12.8 cm, F-stop 2, 0.5 s acquisition time). (b) Excised muscle tissue of theE. coli-infected left leg (left) and theS. aureus-infected right leg (right) of the mouse shown ina. (c) Micro-computed tomography (CT) imaging of the mouse shown inawith bioluminescence (BLI; rainbow scale) and fluorescence (FLI; red–yellow scale) coregistration. A fluorescent signal from the bladder is detectable behind the spine. SeeSupplementary Fig. S4and theSupplementary Movie 1for the separate BLI and FLI images. (d) Fluorescence microscopy of infected muscle tissue. A cluster of vanco-800CW-labelled Gram-positive cocci (that is,S. aureus) is indicated in the right panel (red) and a chain of Gram-negative rods (that is,E. coli) is indicated in the left panel (green). DAPI (4',6-diamidino-2-phenylindole)-stained cell nuclei are labelled green. Scale bar, 10 μm. Vanco-800CW imaging: excitation 710 nm, emission >785 nm; DAPI imaging: excitation 360 nm and emission >458 nm. See alsoSupplementary Fig. S6. Figure 2: In-vivo imaging of bacterial myositis. ( a ) Imaging of a mouse with E. coli (Xen16)-induced myositis in the left hind limb and S. aureus (Xen36)-induced myositis in the right hind limb was performed with the IVIS SpectrumCT Imaging System at 8 and 24 h after intravenous administration of 1.8 mg kg −1 vanco-800CW. Left side: bioluminescence imaging (open filter, field of view (FOV) 12.8 cm, F-stop 1, 30 s acquisition time); right side: fluorescence imaging (excitation 745 nm, emission 840 nm, field of view (FOV) 12.8 cm, F-stop 2, 0.5 s acquisition time). ( b ) Excised muscle tissue of the E. coli- infected left leg (left) and the S. aureus -infected right leg (right) of the mouse shown in a . ( c ) Micro-computed tomography (CT) imaging of the mouse shown in a with bioluminescence (BLI; rainbow scale) and fluorescence (FLI; red–yellow scale) coregistration. A fluorescent signal from the bladder is detectable behind the spine. See Supplementary Fig. S4 and the Supplementary Movie 1 for the separate BLI and FLI images. ( d ) Fluorescence microscopy of infected muscle tissue. A cluster of vanco-800CW-labelled Gram-positive cocci (that is, S. aureus ) is indicated in the right panel (red) and a chain of Gram-negative rods (that is, E. coli ) is indicated in the left panel (green). DAPI (4',6-diamidino-2-phenylindole)-stained cell nuclei are labelled green. Scale bar, 10 μm. Vanco-800CW imaging: excitation 710 nm, emission >785 nm; DAPI imaging: excitation 360 nm and emission >458 nm. See also Supplementary Fig. S6 . Full size image Non-bacterial inflammatory myositis in mice To discriminate a bacterial infection from a sterile foreign body reaction or aseptic inflammation, the fluorescence signal detected after intravenous injection of vanco-800CW in mice with S. aureus -induced myositis ( n =6) was compared with that in mice with sterile myositis induced by implanted Cytodex beads ( n =6). Three of the mice injected with vanco-800CW had S. aureus myositis in the left hind limb, as well as contralateral sterile myositis to reliably compare signals within the same animal. Ex vivo , the muscle tissue with sterile inflammation showed fluorescent signals (1.8 × 10 2 ±0.8 × 10 2 counts) comparable to those of healthy tissue (1.2 × 10 2 ±0.1 × 10 2 counts, P =0.06, not significant; Fig. 3 ). Again, muscle tissue infected with the luciferase-engineered S. aureus emitted significantly higher fluorescence signals (4.1 × 10 2 ±2.6 × 10 2 counts) in comparison with non-infected contralateral healthy muscle tissue ( P =0·008) and tissue with sterile inflammation ( P =0.01; Fig. 3a ). Furthermore, upon correction for background signal, the staphylococcal myositis signal was 2.4-fold stronger than the sterile myositis signal (s.d., 0.15; 95% confidence interval, 2.1–2.7; Fig. 3c ). The presence of sterile inflammation following bead implantation was confirmed by Giemsa staining and light microscopy, which showed accumulation of leukocytes around the beads and absence of leukocytes in healthy muscle tissue ( Fig. 3b ). No bioluminescent bacteria were found in cultures from either the non-infected or sterilely inflamed muscle tissue. 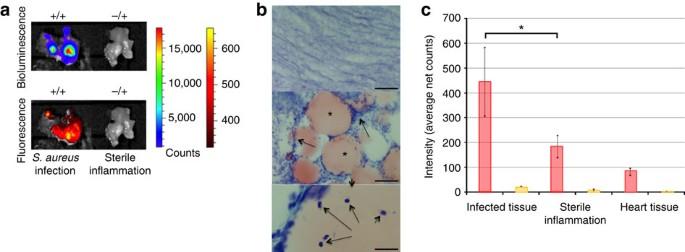Figure 3:In-vivoimaging of bacterial myositis and sterile myositis. (a) Imaging of excised tissue was performed with the IVIS Lumina II. Upper panel, left: bioluminescence detection of bacterial myositis induced withS. aureusXen29 after injection with vanco-800CW (+/+); upper panel, right: bioluminescence detection of sterile myositis after injection with vanco-800CW (−/+); lower panel, left: NIR detection of bacterial myositis induced withS. aureusXen29 after injection of vanco-800CW (+/+); lower panel, right: NIR detection of sterile myositis after injection of vanco-800CW (−/+). Settings for fluorescence measurements: excitation 745 nm, filter ICG; acquisition time 3 s, binning 4, F-stop 2, field of view 12.5 cm; settings for bioluminescence measurements: excitation block, filter open, acquisition time 300 s, binning 4, F-stop 1, FOV 12.5. (b) Confirmation of the presence of leukocytes by microscopy (Giemsa staining). (b, top) non-infected tissue; (b, middleb, bottom) sterile inflammation with Cytodex (*) beads (leukocytes are indicated by black arrows). Scale bars, 200 μm (b, topb, middle) and 20 μm (b, bottom). (c) Quantification ofex-vivofluorescence signals in tissues of bacterial myositis, sterile myositis and heart tissue with the IVIS Lumina II (settings as ina). Bars represent the mean of three mice, error bars display the s.d. Mice treated with vanco-800CW (1 mg kg−1;n=3) are represented by red bars and control non-injected mice (n=3) are represented by yellow bars. Infected tissues yielded a significantly higher signal than sterile inflammation (*P=0·01). Figure 3: In-vivo imaging of bacterial myositis and sterile myositis. ( a ) Imaging of excised tissue was performed with the IVIS Lumina II. Upper panel, left: bioluminescence detection of bacterial myositis induced with S. aureus Xen29 after injection with vanco-800CW (+/+); upper panel, right: bioluminescence detection of sterile myositis after injection with vanco-800CW (−/+); lower panel, left: NIR detection of bacterial myositis induced with S. aureus Xen29 after injection of vanco-800CW (+/+); lower panel, right: NIR detection of sterile myositis after injection of vanco-800CW (−/+). Settings for fluorescence measurements: excitation 745 nm, filter ICG; acquisition time 3 s, binning 4, F-stop 2, field of view 12.5 cm; settings for bioluminescence measurements: excitation block, filter open, acquisition time 300 s, binning 4, F-stop 1, FOV 12.5. ( b ) Confirmation of the presence of leukocytes by microscopy (Giemsa staining). ( b , top) non-infected tissue; ( b , middle b , bottom) sterile inflammation with Cytodex (*) beads (leukocytes are indicated by black arrows). Scale bars, 200 μm ( b , top b , middle) and 20 μm ( b , bottom). ( c ) Quantification of ex-vivo fluorescence signals in tissues of bacterial myositis, sterile myositis and heart tissue with the IVIS Lumina II (settings as in a ). Bars represent the mean of three mice, error bars display the s.d. Mice treated with vanco-800CW (1 mg kg −1 ; n =3) are represented by red bars and control non-injected mice ( n =3) are represented by yellow bars. Infected tissues yielded a significantly higher signal than sterile inflammation (* P =0·01). Full size image Biofilm detection in a human post-mortem implant model To investigate whether vanco-800CW could be employed for non-invasive optical imaging of bacterial biofilms on superficially implanted medical devices, we performed human cadaver TFLI experiments ( n =2) with bacteria-contaminated implants. A three-hole osteosynthesis plate (that is, a one-third tubular plate) was coated with a S. epidermidis biofilm and subsequently incubated with vanco-800CW (plate 1). Plates without biofilm treated with vanco-800CW (plate 2) or plates containing biofilm without vanco-800CW incubation (plate 3) were used as controls. The plates were surgically implanted on the fibula of a human cadaver, followed by standard skin suturing. Subsequently, the lower leg was imaged in both pseudocolour and fluorescence modes with a clinical intraoperative multispectral fluorescence camera system [8] , [16] . A strong fluorescence signal from plate 1 was detected through the skin, whereas neither plate 2 nor plate 3 showed any significant fluorescence signal compared with the background ( Fig. 4a ). Corroborating data were obtained with the IVIS Spectrum imaging system ( Supplementary Fig. S8 ). Subsequent dose–response analyses with vanco-800CW-preincubated S. aureus or S. epidermidis cells spotted onto filter paper and applied to the distal tibia of the left leg of a human cadaver showed that the detection limits for these bacteria were 1.25 × 10 8 or 1.5 × 10 8 CFU mm −2 , respectively ( Fig. 4b ). In this case, the bacteria were covered with about 8 mm of tissue upon skin suturing. 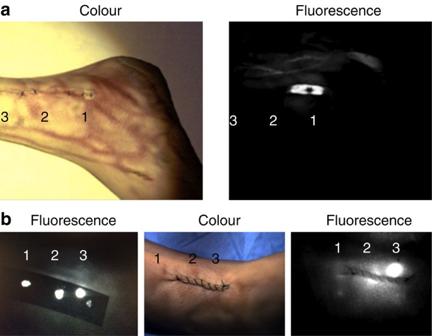Figure 4: Humanpost-mortemimplant model. (a) Osteosynthetic devices were either uncoated (2) or coated with anS. epidermidisbiofilm (1 and 3). Plates 1 and 2 were incubated with vanco-800CW before surgically applying each plate onto the fibula of apost-mortemankle. Subsequent non-invasive examination of the ankle was performed with a clinical multispectral fluorescence camera. (b) Vanco-800CW-labelledS. aureuscells were spotted onto a Whatman paper strip, which was imaged as ina, either before (left fluorescence panel) or after surgical application onto the distal tibia of apost-mortemankle (right fluorescence panel). The tested amounts ofS. aureusapplied to the Whatman paper were: 1, 0.63 × 108CFU mm−2; 2, 1.25 × 108CFU mm−2; 3, 2.5 × 108CFU mm−2. Figure 4: Human post-mortem implant model. ( a ) Osteosynthetic devices were either uncoated (2) or coated with an S. epidermidis biofilm (1 and 3). Plates 1 and 2 were incubated with vanco-800CW before surgically applying each plate onto the fibula of a post-mortem ankle. Subsequent non-invasive examination of the ankle was performed with a clinical multispectral fluorescence camera. ( b ) Vanco-800CW-labelled S. aureus cells were spotted onto a Whatman paper strip, which was imaged as in a , either before (left fluorescence panel) or after surgical application onto the distal tibia of a post-mortem ankle (right fluorescence panel). The tested amounts of S. aureus applied to the Whatman paper were: 1, 0.63 × 10 8 CFU mm −2 ; 2, 1.25 × 10 8 CFU mm −2 ; 3, 2.5 × 10 8 CFU mm −2 . Full size image Detecting bacterial infections in patients remains a challenging clinical problem, with potentially devastating consequences arising from fulminant infections and sepsis. Current non-invasive diagnostic imaging techniques are handicapped by low resolution and specificity due to their shared inability to discriminate between bacterial infection and sterile (non-bacterial) inflammation [4] , [7] . Moreover, these techniques harbour inherent disadvantages that preclude their incorporation in bedside monitoring devices for repetitive clinical application in individual patients. Optical imaging, in particular TFLI imaging, has shown great potential in applications ranging from cancer detection to image-guided surgery [8] , [17] , [18] . Both epi-illumination techniques and novel developments such as opto-acoustics offer highly promising methods for early detection of bacterial infections. Three studies have so far been published, describing in vivo optical imaging of bacterial infections using fluorescent agents [9] , [10] , [11] . Ning et al . [9] used a maltodextrin-IR786 conjugate to detect E. coli , S. aureus , P. aeruginosa and Bacillus subtilis . The conjugate yielded strong bacteria-specific signals in rats after intravenous administration (TBR ratios of 26). The maltodextrin-IR786 probe was also able to discriminate E. coli infection from lipopolysaccharide (LPS)-induced sterile inflammation. However, this probe tends to accumulate only in metabolically active bacteria. Although the authors described biofilm detection using maltodextrin-IR786, this probe might not detect infections containing metabolically inactive bacteria. Furthermore, IR786 has not undergone extensive animal toxicity studies, nor is clinical good manufacturing practice material available. Although maltodextrin is a common food additive, no intravenous data are available for humans. Panizzi et al . [10] reported specific S. aureus endocarditis detection in mice using fluorescently labelled prothrombin (prothrombin-AF680). This agent binds to the staphylococcal coagulase produced by S. aureus on the heart valves, enabling good visualization of S. aureus- induced endocarditis. Prothrombin-AF680 was pharmacologically inactive and no signal was observed in areas of sterile endothelial damage. This suggests that it could be clinically applicable. Nevertheless, prothrombin may not be completely S. aureus -specific, as it is involved in physiological processes, potentially leading to false-positive results [19] . Another potential pitfall of this agent is that staphylococcal coagulase was shown to be expressed only on the borders of mature vegetation, which may yield inadequate signal. Importantly, prothrombin will only reveal coagulase-positive bacteria, which severely limits the spectrum of detectable bacteria. Although there is experience with the intravenous use of prothrombin in humans, AF680 also has not yet undergone extensive animal toxicity studies. Kong et al . [11] demonstrated in vivo detection of Mycobacterium tuberculosis with a ‘smart’ activatable probe. This probe consisted of a β-lactam moiety linking a fluorophore to a fluorescence quencher. After cleavage of the β-lactam ring by β-lactamase, an enzyme endogenously produced by M. tuberculosis and some other bacteria, the fluorophore was separated from the quencher and emitted a signal. Although such smart activatable probes can potentially deliver higher TBRs in optical imaging, not all bacteria produce β-lactamase. In addition, none of the dyes used in this study have undergone extensive animal toxicity studies, which limits their translational use. We have shown here that vanco-800CW enables specific detection of the main Gram-positive bacteria that cause soft tissue and BAIs. Treatment of the latter is most effective during early stages, before extensive biofilm formation has occurred. Therefore, early detection could improve patient outcome and reduce healthcare costs. Vanco-800CW could be ideally used in combination with a multispectral NIR clinical imaging camera as exemplified in our human post-mortem implant experiments. This provides high TBRs owing to reduced tissue autofluorescence and optimal tissue penetration [20] . In-vitro analyses showed highly specific binding of vanco-800CW to all tested clinical BAI isolates of S. aureus and coagulase-negative staphylococci. Variable detection of less common causes of BAI was observed, with good detection of Streptococcus and Dermabacter species and a lesser detection of corynebacteria. As expected, Gram-negative bacteria such as E. coli or P. aeruginosa were not detectable. For S. aureus , the in-vitro limit of detection was estimated to be 2.5 × 10 4 bacteria per mm 3 . Notably, we were able to isolate ~6.4 × 10 7 CFU of S. aureus from ~300–400 mg homogenized tissue taken from the imaged myositic tissue. It has been shown that the majority of soft tissue infections and abscesses caused by Gram-positive cocci contain more than 10 7 CFU ml −1 , corresponding to 10 4 CFU mm −3 (ref. 21 ). Therefore, vanco-800CW should allow detection of the vast majority of clinically relevant Gram-positive bacterial infections in vivo , making it more widely applicable than prothrombin-AF680 or β-lactamase-specific smart activatable probes. The in vivo efficacy of vanco-800CW was demonstrated in a mouse model of myositis induced by bioluminescent S. aureus . The vanco-800CW-specific signal colocalized with the intrinsic bioluminescence of the staphylococcal strain and was able to discriminate S. aureus -induced infection from E. coli -induced infection or sterile inflammation. In terms of biodistribution, strong fluorescence signals were detected in the kidney and urine; a minor signal was detected in the liver. These signals suggested that vanco-800CW was metabolized by the liver into renally excreted products. It is long known that native vancomycin is mainly eliminated from the body by renal excretion [13] . Unconjugated IRDye 800CW is also known to be excreted by the kidneys [14] , [15] . Importantly, the signals emitted from infection sites were clearly distinguishable from the kidney, bladder and liver signals. No significant signal was detected in other organs. As expected, no bowel signal was observed, as vancomycin was unable to penetrate the bowel. Therefore, the gut microbiota should not interfere with imaging of bacterial infections. A post-mortem study using contaminated implants was performed as a clinical simulation to assess the feasibility of BAI detection. S. epidermidis -containing implants stained with vanco-800CW were visible through the cadavers’ skin. Furthermore, vanco-800CW-labelled S. aureus or S. epidermidis cells spotted onto implanted paper strips were detectable at levels of 1·25 × 10 8 or 1·5 × 10 8 CFU mm −2 , respectively. Although this detection limit may seem high, it should be noted that the bacteria were present in a two-dimensional layer covered by ~8 mm of sutured tissue, which mimics the situation in an early-stage biofilm. In a progressive BAI, bacteria will grow in three dimensions, which is likely to be more readily detectable, as was the case in our mouse myositis model. Altogether, our findings imply that detection of early-stage biofilm formation on implants using vanco-800CW is feasible. Nevertheless, limited tissue penetration might pose a challenge in detecting deeper infections arising from hip prosthesis or endocarditis, as the current maximum penetration depth of NIRF is around 1 cm [22] . Another challenge could be that the vascularity around synthetic joint implants may be limited. However, new techniques such as opto-acoustic imaging may allow deeper tissue penetration to a depth of several centimetres and at greater sensitivity, potentially allowing detection of bacterial infections that are seated deeper in the human body [22] . Vancomycin has been extensively applied in the clinic for over 50 years. Using this clinically approved drug as a targeting agent coupled with IRDye 800CW, which has undergone good laboratory practice (GLP) toxicity testing and is being used in a clinical trial (NCT01508572, UMCG), is likely to expedite the translation of the vanco-800CW agent into clinical use after appropriate toxicity testing and good manufacturing practice production according to Good Clinical Practice guidelines [23] . In our mouse model, a strong fluorescence signal emanated from the site of bacterial infection with an intravenous dose of 1 mg kg −1 vanco-800CW, which is tenfold lower than the therapeutic dose in humans (10 mg kg −1 ). Besides, for most clinical imaging indications, only one single bolus injection of the imaging agent will be administered. Accordingly, unwanted side effects such as toxicity or induction of vancomycin resistance in bacteria are unlikely. In summary, we have shown that specific detection of Gram-positive bacterial infections can be achieved with optical imaging using vanco-800CW in vivo in a mouse myositis model. We have also tested vanco-800CW in a human post-mortem BAI implant model, with the intent of developing a novel bedside tool for detecting soft tissue infections and BAI. On the basis of the present findings, we consider vanco-800CW as a very promising clinical optical imaging agent for the detection of Gram-positive bacterial infections. Furthermore, we anticipate that optical imaging will gain a place in day-to-day clinical practice in the fight against severe bacterial infections. Synthesis of vancomycin-IRDye800CW Vancomycin-IRDye800CW (vanco-800CW) was synthesized by an adapted literature procedure [24] . Vancomycin hydrochloride hydrate (3.0 mg, 2.0 μmol; Sigma-Aldrich, St Louis, USA) was added to a solution of IRDye800CW-NHS ester (1.0 mg, 0.86 μmol; LI-COR Biosciences) and N,N -diisopropylethylamine (2.0 μl, 11 μmol; Sigma-Aldrich) in dimethylsulphoxide (200 μl; Sigma-Aldrich). The reaction progress was monitored by analytical reversed-phase HPLC on an Agilent Technologies 1100 Series system with a Polaris C18-A column (100 × 3.0 mm; flow rate 0.5 ml min −1 ; manual injection of 10 μl samples; column temperature 30 °C). HPLC buffer A was 50 mM triethylammonium acetate, 4% acetonitrile, pH 6.0, and HPLC buffer B was 50 mM triethylammonium acetate+80% acetonitrile. The column was equilibrated at 0/100 Buffer B/Buffer A, and the elution gradient was established from 0/100 to 100/0 Buffer B/Buffer A over 10 min (5 min post-time to re-equilibrate column). The monitored wavelengths were 780, 680, 280 and 230 nm. After overnight reaction at ambient temperature, the resulting bioconjugate was purified by preparative reverse-phase HPLC on an Agilent Technologies 1100 Series system with a Zorbax C18 column (250 × 9.6 mm; flow rate 3.0 ml min −1 ; manual injection of 100 μl samples, column temperature 40 °C). The column was equilibrated at 20/80 Buffer B/Buffer A, and the elution gradient was established from 20/80 to 35/65 Buffer B/Buffer A over 15 min (10 min post-time to re-equilibrate column). The monitored wavelengths were 780, 680, 280 and 230 nm. The major peak was collected as two fractions, aliquots of which were checked by ultraviolet–visible spectrometry ( Supplementary Fig. S9 ) and low-resolution mass spectrometry on an Agilent Technologies 1100 Series LC MSD Trap ( Supplementary Fig. S10 ) to determine compound identity, and by analytical HPLC ( Supplementary Fig. S11 ) to determine compound purity. Within the limits of HPLC detection, the final product did not contain any unconjugated dye (detected at 780 nm) or unlabelled vancomycin (detected at 280 nm; Supplementary Fig. S12 ). Fractions containing pure vanco-800CW were pooled, concentrated in vacuo , redissolved in UltraPure water and eluted through Amberlyte IR-120 Ion Exchange Resin (sodium form). The bulk solution of ion-exchanged vanco-800CW was quantified by ultraviolet–visible spectrometry on an Agilent 8453 Series spectrophotometer. The isolated yield for the product was determined to be 1.0 mg (46%, 396 nmol). The product was packaged as 25 nmol aliquots, frozen at −80 °C and lyophilized to afford a green flocculent solid. Ultraviolet–visible (methanol) λ max =778 nm; low-resolution mass spectrometry (electrospray (ES)/ammonium formate), m/z calculated for 24,307 [M—H] − , found 8,106 [M—3H] 3− . Before usage, the vanco-800CW was dissolved in PBS. Biofilm formation The American Type Culture Collection S. epidermidis strain 35984 was plated on agar containing 5% sheep blood and cultured at 35 °C, 5% CO 2 . A colony was transferred to Tryptic soy broth (TSB)+2.5% glucose and cells were cultivated at 35 °C for 2 days under shaking. Finally, a 200-fold dilution of the S. epidermidis suspension was incubated with an osteosynthetic device (that is, one-third tubular plate) in TSB+2.5% glucose medium overnight at 35 °C. Incubation with vancomycin-IRDye800CW Bacteria or biofilm-bearing biomaterials were incubated with TSB+2·5% glucose medium containing vanco-800CW (0.14 nmol ml −1 ) for 2 h at 35 °C, 5% CO 2 . Subsequently, the incubated material was washed twice with PBS. For bacterial suspensions, the materials were centrifuged (8 min at 16,873 relative centrifugal force) and the supernatants were removed. The pellets were resuspended in PBS or TSB. In-vitro imaging analyses were performed using an IVIS Spectrum (Caliper LS, Hopkinton, MA, USA). Clinical isolates Samples of bacterial infections related to orthopaedic biomaterial, occurring over 1 year at the UMCG, were collected (2010–2011, 32 patients with 150 isolates). A selection of variably occurring species was prepared to mimic microbial populations associated with BAIs. Selected isolates (38 from 19 different patients) were thawed and cultured on blood agar plates (5% sheep blood) for 3 days at 35 °C, 5% CO 2 . Suspensions at an optical density of 3.5–4.2 McFarland were prepared, incubated with vanco-800CW and washed twice with PBS. Samples were centrifuged and pellets were resuspended in 200 μl PBS and pipetted into 96-well plates (BD Falcon, black). Imaging was performed with the IVIS Spectrum, using the settings specified in Figure S1. The experiment was performed twice in duplicate. Limit of bacterial detection To determine the limit of bacterial detection, a clinical isolate of S. aureus was suspended in TSB+2·5% glucose medium (4 McFarland in 2 ml). The suspension was incubated with vanco-800CW, washed twice with PBS and resuspended in PBS. Numbers of bacteria were calculated using a cell counting chamber (Bürker), at a 200-fold dilution and optical enhancement with safranin 0·1%. Counting was done independently by two researchers. A series of dilutions in 180 μl PBS was prepared in black 96-well plates. The experiment was performed thrice in duplicate with non-treated S. aureus as a negative control. Imaging analysis was performed with the IVIS Spectrum. After analysis, incubated S. aureus and non-treated S. aureus were plated on blood agar and cultured overnight at 35 °C, 5% CO 2 , to determine whether vanco-800CW at the used dosage would impair viability. Mouse experiments Experimental animal studies shown in Fig. 3 and Supplementary Figs S2, S5, S7 and S9 were performed at the Institut für Molekulare Infektionsbiologie, Universität Würzburg, Würzburg, Germany. These studies were approved by the Committee on the Ethics of Animal Experiments of the government of Lower Franconia, Germany (55.2–2531.01-06/12), and were performed in strict accordance with the German animal protection law. Experimental animal studies shown in Fig. 2 , Supplementary Figs S3, S4 and S6 , and Supplementary Movie 1 were performed at the PerkinElmer facility in Alameda, CA, USA. These studies were approved under the IACUC protocol number 003 (expiry date 1 August 2014). They were carried out by qualified personnel with strict compliance to rules and regulations for the PerkinElmer facility in Alameda, to ensure that all animals were humanely treated. Bioluminescent S. aureus (Xen29, Caliper LS) was used to induce a hind limb myositis in 12 Naval Medical Research Institute (NMRI) mice [25] . The applied dose of 5 × 10 7 CFU per injection was the minimum dose at which a readily detectable myositis developed ( Supplementary Fig. S13 ). Two days post infection, vanco-800CW was intravenously administered (0·1–5 mg kg −1 ) to six infected mice and six non-infected mice. After 24 h, the 12 infected and six non-infected mice were killed and imaged with an IVIS Lumina II (Caliper LS) to detect fluorescence and bacterial bioluminescence. In co-infection experiments, NMRI mice were infected with bioluminescent S. aureus (Xen36) and E. coli (Xen16; Caliper LS) at 5 × 10 7 CFU per injection. Low-dose micro-computed tomography (CT) was performed with a Quantum FX microCT Imaging System within the IVIS SpectrumCT (Caliper LS). Infected muscle tissue was excised and subsequently imaged with the IVIS Lumina II or the IVIS SpectrumCT. Infected tissue was homogenized and cultured or stored at −80 °C. Bacterial presence in excised tissue was visualized either by fluorescence microscopy or by Giemsa staining and light microscopy. For NIRF microscopy, tissues were fixed overnight with 4% paraformaldehyde in PBS (pH 7.5) and washed thrice in PBS (10 min), twice in 70% ethanol (1 h) and twice in 95% ethanol (1 h). Fixed tissue was embedded in paraffin and 5-μm-thick sections were cut. Deparaffinization and rehydration of tissue slides were performed by washing in xylene (5 min, thrice), 100% ethanol (2 min, twice), 96% ethanol (2 min), 80% ethanol (2 min), 70% ethanol (2 min), 50% ethanol (2 min), distilled water (2 min) and PBS (5 min). Vectashield mounting medium (Vector Laboratories, Burlingame, CA, USA) with DAPI (4',6-diamidino-2-phenylindole) was added and a coverslip was placed. Fluorescence imaging was performed with the Nuance EX multispectral charge-coupled device camera (PerkinElmer, Hopkinton) and an Eclipse E400 microscope (Nikon, Japan). For Giemsa staining, frozen tissue sections were made (6 μm thickness) and mounted on slides. The sections were fixed in methanol for 1 min, rinsed with water, treated with 2·5% Giemsa dilution in PBS for 30 min and rinsed with water. Fluorescent in situ hybridization with an eubacterial (EUB)–fluorescein isothiocyanate probe was performed to confirm the presence of bacteria [26] . Briefly, sections were fixed with methanol and dried on a hot plate. Next, sections were treated with permeabilization buffer, rinsed with methanol and dried on a hot plate. The EUB–fluorescein isothiocyanate probe dissolved in urea buffer (10 ng μl −1 ) was added to the sections, followed by incubation for 20 min on a hot plate [27] . The sections were washed twice, covered with Vectashield (Vector Laboratories) and coverslipped. Analysis was performed using fluorescence microscopy (Leica CTR5500; Leica Microsystems BV, Rijswijk, The Netherlands). To induce a sterile inflammation, Cytodex beads (1 mg in 50 μl; Sigma-Aldrich) were injected in the upper leg muscle of four NMRI mice [28] . Vanco-800CW was intravenously administered (1 mg kg −1 ) to two mice. To compare the sterile inflammation with bacterial myositis, S. aureus (Xen29) was introduced to the left hind limbs of six mice, whereas Cytodex beads were introduced into their contralateral right hind limbs. Three mice were treated with vanco-800CW (1 mg kg −1 ) and compared with three negative controls. Imaging was performed with the IVIS Lumina II, and tissues were collected as described above. Frozen tissue sections were made and Giemsa-stained to confirm leukocyte infiltration. To determine the staphylococcal burden of infected muscles, tissue was aseptically collected at indicated time points and homogenized in 2 ml of sterile PBS using Dispomix (Bio-Budget Technologies GmbH, Krefeld, Germany). Serial dilutions of the homogenates were cultured on mannitol salt–phenol red agar plates for at least 48 h at 37 °C. Colonies were counted and staphylococcal burden was calculated as total CFU/excised tissue. Bioluminescence signal was determined using the IVIS Lumina II. Human post-mortem implant model Biofilms were formed on two osteosynthetic devices (one-third tubular plates) by incubation with S. epidermidis ATCC 35984. Subsequently, biofilm-coated plates and uncoated control plates were incubated with vanco-800CW as mentioned above and washed twice with PBS. The three differently treated osteosynthetic devices were implanted on the distal fibula in a human cadaver ankle and the skin was subsequently sutured (Ethilon 3-0, Ethicon Somerville, NJ, USA). Imaging was performed using an intraoperative clinical multispectral fluorescence camera (T 3 -imaging system, SurgOptix BV, Groningen, The Netherlands) and the IVIS Spectrum [8] , [16] . The experiment was performed twice with the lower legs of two human cadavers. For dose–response measurements, dilution series of vanco-800CW-treated S. aureus SH1000 or S. epidermidis ATCC 35984 were spotted on Whatman 3MM paper strips (ranging from 2.5 × 10 4 to 2.5 × 10 8 CFU mm −2 , or from 1.5 × 10 4 to 1.5 × 10 8 CFU mm −2 , respectively). These were subsequently implanted on the medial site of the distal tibia in a human cadaver ankle, and imaging was performed with the T 3 intraoperative clinical multispectral fluorescence camera. The post-mortem experiments were conducted according to institutional guidelines with prior approval from the scientific review committee of the Skills Center of the University Medical Center Groningen, The Netherlands. All individuals involved in the human post-mortem studies have provided informed written consent for the use of their bodies for scientific research and teaching. Software Results obtained with the IVIS systems were analysed with Living Image 4·2 (Caliper LS). Optimal detection limits were set to the lowest signal at which the positive signal was effortlessly discriminated from negative controls. Signal intensity was determined by drawing regions of interests and measuring average counts in these regions. The signal was corrected for background by subtracting the background signal from the signal of interest, referred to in the text as net counts. Statistics Fluorescence imaging data derived by the IVIS systems are expressed in counts as mean±2 s.d. in the regions of interest. For determining statistical relationships among bacterial infection, sterile inflammation or negative controls, either the paired or unpaired two-sample Student’s t -test ( P <0.05) was used. How to cite this article: van Oosten, M. et al . Real-time in vivo imaging of invasive- and biomaterial-associated bacterial infections using fluorescently labelled vancomycin. Nat. Commun. 4:2584 doi: 10.1038/ncomms3584 (2013).